Formin mDia1 senses and generates mechanical forces on actin filaments Cytoskeleton assembly is instrumental in the regulation of biological functions by physical forces. In a number of key cellular processes, actin filaments elongated by formins such as mDia are subject to mechanical tension, yet how mechanical forces modulate the assembly of actin filaments is an open question. Here, using the viscous drag of a microfluidic flow, we apply calibrated piconewton pulling forces to individual actin filaments that are being elongated at their barbed end by surface-anchored mDia1 proteins. We show that mDia1 is mechanosensitive and that the elongation rate of filaments is increased up to two-fold by the application of a pulling force. We also show that mDia1 is able to track a depolymerizing barbed end in spite of an opposing pulling force, which means that mDia1 can efficiently put actin filaments under mechanical tension. Our findings suggest that formin function in cells is tightly coupled to the mechanical activity of other machineries. Physical forces participate in the regulation of biological functions, from embryonic development to adult physiology, and are key factors in numerous pathological processes [1] . Individual cells are sensitive to their mechanical environment, which can be used to steer stem cell differentiation [2] . Single-molecule approaches have provided insight into some molecular mechanisms responsible for the conversion of physical forces into biochemical signals. For example, talin, a protein involved in mechano-transduction at focal adhesions, exposes buried vinculin interaction sites when it is stretched by forces of tens of piconewtons [3] . Molecular motors that convert the energy from ATP hydrolysis into mechanical movement along filament tracks are also sensitive to applied forces in the piconewton range, and have been studied with extreme accuracy [4] , [5] . In stark contrast, nearly nothing is known about the regulation of cytoskeletal filament assembly by mechanical forces, besides the slowing down of polymerization by an opposing obstacle—an effect observed more clearly for microtubules [6] than actin filaments [7] , which are too flexible to work individually. Evidence of a mechanism where a mechanical force modulates the elongation of individual actin filaments is still missing. Formins elongate actin filaments while remaining processively attached to their growing barbed ends [8] , [9] . They are responsible for the rapid generation of long actin cables which form the backbone of key cellular substructures such as filopodia [10] , stress fibres [11] and cytokinetic rings [12] , [13] . Formin elongation has been proposed to be mechano-sensitive [14] , as the two protomers of the FH2 (Formin Homology domain 2) dimer translocate in a rotating stair-step fashion to track the elongating barbed end [15] , [16] . From a physiological perspective, the regulation of formin activity by mechanical forces would have a central role in numerous situations where formin-elongated filaments are eventually put under tension, for example, during filopodia retraction or cytokinetic ring contraction. The aim of the present work is to establish how a formin responds to the application of mechanical tension on the filament that it is elongating. We use microfluidics to apply piconewton pulling forces to individual actin filaments elongated by surface-anchored formin mDia1, and show that their elongation rate can thus be increased up to two-fold. This increase in elongation rate can be understood by considering that the pulling force favours the ‘open’ conformation of the FH2 dimer, in which an additional actin subunit can be added at the filament barbed end. The mechanical response of formin mDia1 is the same whether the pulling force is applied at the N-terminal side of the FH1 domain or at the C-terminal side of the FH2 domain. We also show that formin mDia1 remains processively bound to the barbed end of a depolymerizing filament which is being pulled on, and that the pulling force slows down depolymerization. This result implies that formins can put actin filaments under tension. Applying forces to individual filaments with microfluidics In order to apply pulling forces to individual filaments, we have taken advantage of a yet unexploited mechanical feature of our recently developed microfluidics setup [17] , [18] . In this experimental configuration, filaments grow anchored by one end to the glass coverslip surface at the bottom of a flow chamber. The filaments are aligned and maintained close to the coverslip surface by the flow ( Fig. 1b ). The viscous drag exerted by the flowing liquid on the anchored filament results in a pulling force, which is maximal at the anchoring point. Using a bead in an optical trap to measure this force, we have verified that it was proportional to the local fluid velocity times the length of the filament, and thereby determined the longitudinal friction coefficient for an actin filament ( Fig. 1a , Methods). 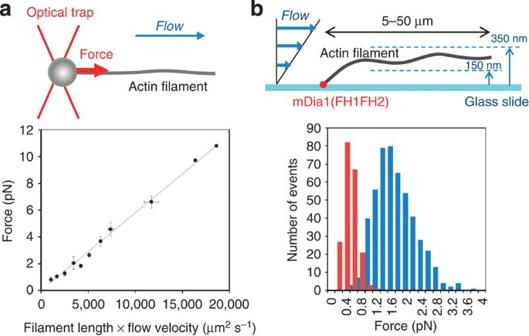Figure 1: Pulling on actin filaments with the viscous drag of a flowing fluid. (a) The force exerted by the flowing fluid on an actin filament is measured with a microbead in an optical trap, a few micrometres above the surface. Data points and error bars show the averages and s.d. of 47 measurements, performed with different filament lengths and different flow velocities. (b) Filaments anchored to the bottom of the microfluidic chamber fluctuate around an average position located 250 nm above the surface, resulting in rapid fluctuations of the force exerted on the anchoring point. Histograms show the force distributions for a 14-μm long filament in a flow velocity gradient of 194 s−1(red bars, force=0.40±0.16 pN) and for a 20-μm long filament in a flow velocity gradient of 565 s−1(blue bars, force=1.63±0.53 pN). Figure 1: Pulling on actin filaments with the viscous drag of a flowing fluid. ( a ) The force exerted by the flowing fluid on an actin filament is measured with a microbead in an optical trap, a few micrometres above the surface. Data points and error bars show the averages and s.d. of 47 measurements, performed with different filament lengths and different flow velocities. ( b ) Filaments anchored to the bottom of the microfluidic chamber fluctuate around an average position located 250 nm above the surface, resulting in rapid fluctuations of the force exerted on the anchoring point. Histograms show the force distributions for a 14-μm long filament in a flow velocity gradient of 194 s −1 (red bars, force=0.40±0.16 pN) and for a 20-μm long filament in a flow velocity gradient of 565 s −1 (blue bars, force=1.63±0.53 pN). Full size image Filaments anchored at the bottom of the flow cell are in a region where the flow velocity increases linearly with distance away from the surface ( Supplementary Fig. S1 ). As the anchored filament fluctuates in the flowing fluid, it explores different distances away from the surface. Using Total Internal Reflection Fluorescence (TIRF) microscopy with a calibrated penetration depth ( Supplementary Fig. S2 ) we have measured the contour profile of individual filaments, which fluctuate around an average position 250 nm above the surface for the range of flow velocities and filament lengths used in this work ( Supplementary Fig. S3 ). The force exerted on the anchoring point is computed by integrating the viscous drag over the whole-filament contour, which experiences different local flow velocities as it explores different distances above the surface. Within a 10% error, the average force is equal to the viscous drag the filament would experience if it remained entirely 250 nm above the surface. The force fluctuates within ±30% of its average value, at a frequency far superior to that of data acquisition ( Fig. 1b , Supplementary Fig. S3 , Methods). When a filament grows from a surface-anchored spectrin-actin seed, no significant force is exerted on a formin interacting with its freely growing barbed end ( Fig. 2a ). In this situation, as in the absence of formin [17] , the flow velocity has no impact on the elongation rate. 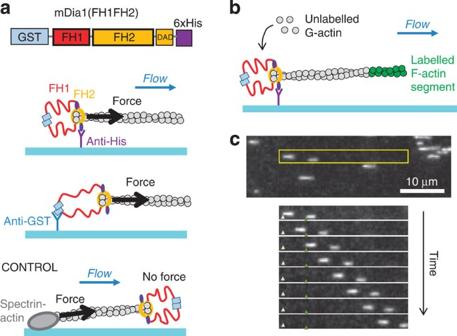Figure 2: Applying forces to surface-anchored formins as they elongate actin filaments. (a) The mDia1(FH1FH2) construct comprises the DAD domain, as well as a C-terminal His-tag and an N-terminal GST-tag. The use of biotinylated antibodies and a streptavidin-coated surface allows the specific anchoring of mDia1(FH1FH2) dimers by their FH1 or FH2 domains. Control experiments where the formin feels no force are performed by growing filaments from surface-anchored spectrin-actin seeds. (b) An anchored mDia1(FH1FH2) elongates a filament from its barbed end using unlabelled monomers, following a brief elongation from fluorescently labelled actin, which formed the fluorescent segment visible at the pointed end. (c) Epifluorescence image of the situation sketched in (b) with 1 μM unlabelled ATP-actin and 4 μM profilin. The time sequence corresponds to the area indicated by the yellow frame in the larger image, and toSupplementary Movie 1. The interval between two images is 20 s. The triangles indicate the location of two anchored mDia1(FH1FH2) dimers. The flow velocity 250 nm above the surface is 101 μm s−1. Figure 2: Applying forces to surface-anchored formins as they elongate actin filaments. ( a ) The mDia1(FH1FH2) construct comprises the DAD domain, as well as a C-terminal His-tag and an N-terminal GST-tag. The use of biotinylated antibodies and a streptavidin-coated surface allows the specific anchoring of mDia1(FH1FH2) dimers by their FH1 or FH2 domains. Control experiments where the formin feels no force are performed by growing filaments from surface-anchored spectrin-actin seeds. ( b ) An anchored mDia1(FH1FH2) elongates a filament from its barbed end using unlabelled monomers, following a brief elongation from fluorescently labelled actin, which formed the fluorescent segment visible at the pointed end. ( c ) Epifluorescence image of the situation sketched in ( b ) with 1 μM unlabelled ATP-actin and 4 μM profilin. The time sequence corresponds to the area indicated by the yellow frame in the larger image, and to Supplementary Movie 1 . The interval between two images is 20 s. The triangles indicate the location of two anchored mDia1(FH1FH2) dimers. The flow velocity 250 nm above the surface is 101 μm s −1 . Full size image Here, we elongate filaments from surface-anchored formins on which we thus exert a pulling force. We have used a formin construct mDia1(FH1FH2), which comprises the functional FH1 and FH2 domains, as well as the DAD domain which has no impact on filament elongation [19] , an N-terminal GST tag and a C-terminal His tag ( Fig. 2 ). Proper passivation of the coverslip surface and functionalization with streptavidin ensured the specific anchoring of either the N-ter-FH1 or the C-ter-FH2 domain of mDia1(FH1FH2) pre-incubated with biotinylated anti-GST or anti-His antibodies ( Fig. 2 ), without affecting their activity (Methods). As fluorescent labelling can give rise to unexpected artifacts [20] , we monitor the elongation of filaments from unlabelled actin monomers, by first nucleating and elongating fluorescent filament segments, and subsequently flowing a solution of unlabelled actin in the microchamber ( Fig. 2b ). Elongation is monitored by tracking the position of the fluorescent filament segment as it moves away from the anchored mDia1(FH1FH2). Pulling forces accelerate elongation by formin mDia1 At a given flow rate, the force exerted on the anchored mDia1(FH1FH2) increases progressively as the filament elongates, and the elongation rate increases with this force ( Fig. 3 ). The pulling force can also be varied rapidly by changing the flow rate. The relation between force and elongation rate does not depend on the method by which the force is varied, and the elongation rate drops upon a decrease of the pulling force ( Fig. 3a and Supplementary Fig. S4 ). Forces hence modulate formin activity in a reversible fashion. 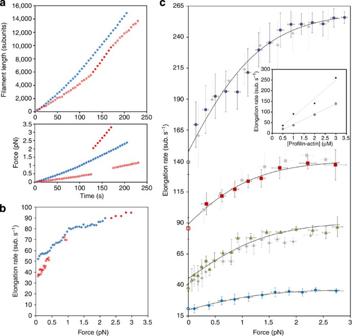Figure 3: Pulling forces increase the elongation rate of filaments from mDia1(FH1FH2). (a) Traces for two different filaments, elongating from 1 μM ATP-actin and 4 μM profilin. One filament is exposed to a flow velocity of 101 μm s−1(blue diamonds) while the other is exposed to a flow velocity of 54 μm s−1(red open circles) with a temporary increase to 215 μm s−1(red bullets). Each actin subunit contributes to 2.7 nm of the filament length. (b) Resulting elongation rate versus force for each filament. (c) Average data from traces of 8–14 filaments for each profilin–actin concentration: 0.5 μM (blue diamonds,n=9 filaments), 1 μM (triangles,n=8), 2 μM (squares,n=14) and 3 μM (bullets,n=11), each with a 3-μM excess of profilin. Error bars are s.d. All data were obtained with mDia1(FH1FH2) anchored by the FH2 domain, except grey data points where the anchor was on the FH1 domain. Open symbols correspond to control experiments with unanchored formins at the barbed end of filaments grown from anchored spectrin-actin seeds. Lines are fits of the data by equation (2), performed withp0and the plateau velocitykon(C−Cc) as free parameters for each set of data. Inset: plot of the resulting plateau values (black symbols) at high force, as a function of profilin–actin concentration, compared with elongation rates in the absence of force (open symbols). Lines are linear fits. Figure 3: Pulling forces increase the elongation rate of filaments from mDia1(FH1FH2). ( a ) Traces for two different filaments, elongating from 1 μM ATP-actin and 4 μM profilin. One filament is exposed to a flow velocity of 101 μm s −1 (blue diamonds) while the other is exposed to a flow velocity of 54 μm s −1 (red open circles) with a temporary increase to 215 μm s −1 (red bullets). Each actin subunit contributes to 2.7 nm of the filament length. ( b ) Resulting elongation rate versus force for each filament. ( c ) Average data from traces of 8–14 filaments for each profilin–actin concentration: 0.5 μM (blue diamonds, n =9 filaments), 1 μM (triangles, n =8), 2 μM (squares, n =14) and 3 μM (bullets, n =11), each with a 3-μM excess of profilin. Error bars are s.d. All data were obtained with mDia1(FH1FH2) anchored by the FH2 domain, except grey data points where the anchor was on the FH1 domain. Open symbols correspond to control experiments with unanchored formins at the barbed end of filaments grown from anchored spectrin-actin seeds. Lines are fits of the data by equation (2), performed with p 0 and the plateau velocity k on ( C − C c ) as free parameters for each set of data. Inset: plot of the resulting plateau values (black symbols) at high force, as a function of profilin–actin concentration, compared with elongation rates in the absence of force (open symbols). Lines are linear fits. Full size image To understand what causes this increase in elongation rate upon the application of a pulling force, we have measured this effect at different profilin–actin concentrations ( Fig. 3c ). Pulling forces increase the elongation rate to a plateau value that is roughly twice the value in the absence of force, with a half-effect reached for a force of ~0.6 pN. The same behaviour is observed whether mDia1(FH1FH2) is anchored via anti-His antibodies, thereby pulling on the FH2 domain alone, or via anti-GST antibodies, thereby pulling on the FH1 domain as well ( Figs 2a , 3c ). The pulling force exerted on the FH2 dimer should favour its translocation [14] . The linear increase of elongation rate with profilin–actin concentration in the absence of force ( Fig. 3c inset) indicates that the translocation of the FH2 dimer is not rate-limiting and that we can consider the FH2 dimer to be in rapid equilibrium between a ‘closed’ conformation, in which no subunit can be added, and an ‘open’ conformation, in which subunits can be added with rate constant k on to the barbed end [15] , [21] ( Fig. 4 ). The elongation rate can be written as v elong = p 0 k on ( C−C c ), where C is the profilin–actin concentration, C c is the critical concentration and p 0 is the probability to find the FH2 dimer in the open conformation. 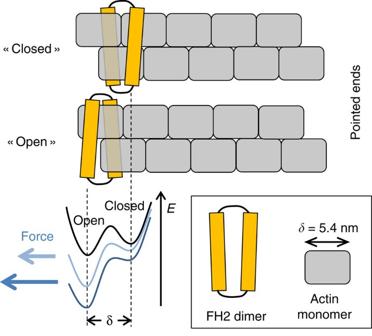Figure 4: Schematic representation of FH2 dimer translocation at the barbed end of an actin filament. The filament barbed end is in a non-polymerizing state when the FH2 dimer is in the ‘closed’ conformation, while it can bind an actin monomer (not shown) when the FH2 dimer is in the ‘open’ conformation15. When analysing filament depolymerization, we consider that the FH2 dimer in the ‘open’ conformation prevents the departure of the terminal actin subunit from the barbed end. Applying a pulling force tilts the energy landscape of the FH2 dimer at the barbed end, favouring the ‘open’ conformation. In the frame of reference of the microchamber, the FH2 dimer is in a fixed location and the filament is displaced as it elongates or depolymerizes. Based on a simple description of translocation using transition state theory [22] , [23] , we can write that upon application of a pulling force F , the probability p 0 becomes Figure 4: Schematic representation of FH2 dimer translocation at the barbed end of an actin filament. The filament barbed end is in a non-polymerizing state when the FH2 dimer is in the ‘closed’ conformation, while it can bind an actin monomer (not shown) when the FH2 dimer is in the ‘open’ conformation [15] . When analysing filament depolymerization, we consider that the FH2 dimer in the ‘open’ conformation prevents the departure of the terminal actin subunit from the barbed end. Applying a pulling force tilts the energy landscape of the FH2 dimer at the barbed end, favouring the ‘open’ conformation. In the frame of reference of the microchamber, the FH2 dimer is in a fixed location and the filament is displaced as it elongates or depolymerizes. Full size image where δ =5.4 nm is the actin monomer size, k is Boltzmann’s constant and T is temperature. The elongation rate can hence be written as Fits of our data by this simple model, with p 0 and k on (C−C c ) as free parameters for each curve, are shown in Fig. 3c . We can hence interpret our results by considering that a pulling force accelerates filament elongation by favouring the open conformation of the FH2 dimer. In the conditions of our measurements (that is, with a 3 μM excess of profilin), we find k on =84.8 μM −1 s −1 and C c =0.07 μM ( Fig. 3c , inset). In the absence of force, the FH2 dimer is in the open conformation only 56% of the time ( p 0 =0.56±0.06), resulting in a slower elongation, with an ‘apparent on-rate’ of 48.1 μM −1 s −1 . Formin mDia1 generates tension on depolymerizing filaments Recent work on individual actin filaments has shown that mDia1(FH1FH2) is able to track a depolymerizing barbed end [16] . Using our control configuration, where no force is applied to mDia1(FH1FH2), we confirm this observation. We have previously reported that free barbed ends depolymerize faster in the presence of profilin [17] and we now show that this effect is further amplified by the presence of mDia1(FH1FH2) at the barbed end ( Fig. 5b ). This effect is reminiscent of the acceleration of barbed end elongation from profilin–actin by formins. Future experiments should reveal whether this effect is due to the action of FH1 alone or also involves an alteration of the barbed end by the FH2 dimer. 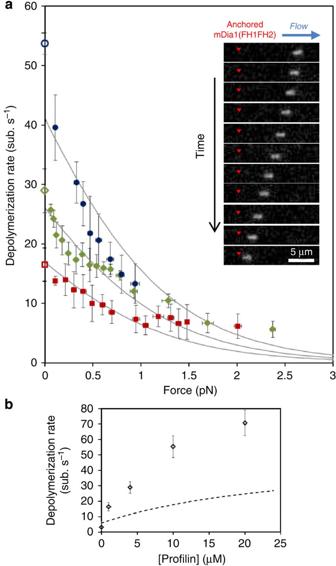Figure 5: mDia1(FH1FH2) can generate piconewton pulling forces on depolymerizing actin filaments. (a) Effect of force on the depolymerization rate of ADP-actin filaments bound to mDia1(FH1FH2) anchored by their FH2 domain, in the presence of 1 μM (red squares,n=4 filaments), 4 μM (green diamonds,n=8) and 10 μM (blue bullets,n=4) profilin. Open symbols correspond to control experiments with unanchored formins at the barbed end of filaments grown from anchored spectrin-actin seeds. Error bars are s.d.. Lines are fit of the data by equation (3). Inset: epifluorescence time sequence of an ADP-actin filament bound to a surface-anchored mDia1(FH1FH2), depolymerizing in the presence of 4 μM profilin, while exposed to a flow velocity of 52 μm s−1(Supplementary Movie 2). Only the fluorescent segment near the pointed end is visible. The interval between images is 20 s. (b) Depolymerization rate of ADP-actin filament barbed ends by mDia1(FH1FH2) in the absence of force, as a function of profilin concentration (data points), compared with the depolymerization rate without mDia1 (dashed line, determined in Jegouet al.17). Figure 5: mDia1(FH1FH2) can generate piconewton pulling forces on depolymerizing actin filaments. ( a ) Effect of force on the depolymerization rate of ADP-actin filaments bound to mDia1(FH1FH2) anchored by their FH2 domain, in the presence of 1 μM (red squares, n =4 filaments), 4 μM (green diamonds, n =8) and 10 μM (blue bullets, n =4) profilin. Open symbols correspond to control experiments with unanchored formins at the barbed end of filaments grown from anchored spectrin-actin seeds. Error bars are s.d.. Lines are fit of the data by equation (3). Inset: epifluorescence time sequence of an ADP-actin filament bound to a surface-anchored mDia1(FH1FH2), depolymerizing in the presence of 4 μM profilin, while exposed to a flow velocity of 52 μm s −1 ( Supplementary Movie 2 ). Only the fluorescent segment near the pointed end is visible. The interval between images is 20 s. ( b ) Depolymerization rate of ADP-actin filament barbed ends by mDia1(FH1FH2) in the absence of force, as a function of profilin concentration (data points), compared with the depolymerization rate without mDia1 (dashed line, determined in Jegou et al. [17] ). Full size image The fact that a formin can track a depolymerizing barbed end suggests that it could perhaps generate pulling forces on the disassembling filament. To address this question, we have triggered the depolymerization of filaments under mechanical force in our microfluidic setup, by flowing in a solution of profilin. We observe that mDia1(FH1FH2) remains bound to the depolymerizing filament, pulling it upstream against piconewton forces, thus showing that formins are able to generate mechanical forces ( Fig. 5 ). This activity was observed on filaments elongated from ATP-actin and depolymerized in standard F-buffer ( Supplementary Fig. S5 ) as well as filaments elongated from ADP-actin and depolymerized in ATP-free buffer ( Fig. 5 ). To further characterize the mechanical response of mDia1(FH1FH2) as a force-generating motor, we have measured the depolymerization rate of ADP-actin filaments against different loads ( Fig. 5 ). We find that a pulling force exerted on the filaments slows down depolymerization. As for elongation experiments ( Fig. 3 ), we have verified that this effect is reversible, and that the depolymerization rates measured against a very low pulling force are similar to control measurements in the absence of force. Following a similar reasoning as for elongation, we can assume that the terminal actin subunit can depart from the barbed end, with a rate constant k off , only when the FH2 dimer is in the ‘closed’ conformation ( Fig. 4 ). The depolymerization rate can then be written as Fits of our data by this simple model, with p 0 =0.56 (determined by the fits of the elongation data by equation (2)), δ =5.4 nm, and leaving k off as a free parameter for each curve, are shown in Fig. 5 . As for elongation, the interpretation here is that the pulling force favours the ‘open’ conformation of the FH2 dimer. This simple two-state model accounts for the observed force-induced decrease of the depolymerization rate, but misses some of its features. For instance, our data indicate that the force-depolymerization profile becomes less sensitive to profilin concentration as force increases, more drastically than what is computed theoretically, suggesting that the interaction of profilin with the formin-bound barbed end may also be affected by force. Also, the computed depolymerization rates are nearly zero at 3 pN, whereas the experimental data seem to indicate a higher stall force. Indeed, our experimental data show that depolymerization remains significant for forces as high as 2.4 pN. Under these conditions, mDia1 produces a mechanical work of ~13 pN nm≈3.2 kT for every departing actin subunit. To describe the conformation changes of the FH2 dimer during filament elongation, one can use the ‘gating factor’, which is defined as the ratio of the elongation rate of barbed ends with and without FH2, in the absence of profilin [21] . The gating factor can be written as , where and are the monomer on-rate constants in the presence and absence of an FH2 dimer, respectively. For mDia1, the gating factor is of the order of 0.9. If we assume that the translocation of the FH2 domain is not affected by profilin, our estimated value of =0.56 leads to . Our results therefore indicate that the mDia1 FH2 dimer, when present at the filament barbed end in the open conformation, increases the on-rate constant of actin monomers by 60%. Formin mechano-sensitivity has been proposed by Kozlov and Bershadsky [14] to stem from FH2 elasticity. We could not fit our data with this model where an activation energy, associated to a rate-limiting formin deformation step (translocation), is reduced by the pulling force. Nonetheless, it is possible that formin elasticity contributes to the energy landscape sketched in Fig. 4 . The FH1 domain is often presented as a flexible chain that captures and delivers profilin–actin to the barbed end [21] . The FH1 domain of mDia1 comprises n =14 polyproline domains of length d ≈3 nm, separated by linkers. Assuming these linkers are flexible, we can model the FH1 domain as a flexible chain, with an ‘entropic spring’ stiffness of 3 kT / nd 2 ≈0.1 pN nm −1 . A 1 pN force should then be able to stretch the FH1 domain, keeping its extremities 10 nm apart. This is a significant constraint on the possible conformations that the FH1 chain, which has a full contour length of about 42 nm, is able to explore. If the FH1 domain delivers profilin–actin to the barbed end by taking advantage of its flexibility to rapidly explore different conformations, the elongation rate of mDia1(FH1FH2)-bound filaments should decrease drastically when piconewton forces are applied on the FH1 domain, compared with the situation where the pulling force is applied to the FH2 domain alone. Beyond this ‘capture and delivery’ mechanism, it seems likely that during FH1-assisted elongation the newly added actin subunit is transiently bound to profilin-FH1 and to the FH2-filament barbed end simultaneously. This configuration should become extremely difficult to achieve when polyproline regions of the FH1 domain are pulled away from the barbed end by pN forces. Our results therefore indicate that the flexible FH1 domain is able to remain in the vicinity of the FH2 dimer and the barbed end, in spite of a pulling force applied on its N-terminal extremity. This could be achieved by interactions of FH1 polyproline helices with FH2 alpha-helices. [24] Such a connection between the FH1 and FH2 domains could lead to a situation where the N-terminal region of the FH1 domain is maintained close to the C-terminal region of the FH2 domain, and pulling on one or the other would have very similar consequences. Elucidating the detailed function of FH1 in rapid processive growth from profilin–actin will require the combination of mechanical experiments like the present ones and of biochemical approaches [25] , which by themselves have not brought definite answers. The generation of force by proteins tracking depolymerizing filament ends has been proposed theoretically [26] , [27] but has only been observed so far for microtubules, with either depolymerizing motors [28] or ‘passive couplers’ [29] . Formin mDia1 bears more similarities with the latter as it does not hydrolyse ATP, and converts energy from actin conformational changes into mechanical work. However, even though mDia1 does not directly induce depolymerization, it largely amplifies the depolymerizing action of profilin ( Fig. 5b ). The pulling forces that we apply to the filaments also detach formins from the surface ( Supplementary Fig. S6 ), thereby limiting the collection of data at high forces, and precluding the study of the force dependence of formin departure from the barbed end (processivity). With a stronger anchoring of formins to the surface, future experiments should allow the study of the release of the filament by mDia1(FH1FH2) and provide accurate measurements of the stall force of depolymerization. Nonetheless, the pulling forces generated by mDia1(FH1FH2) that we measure are large enough to play a role in cells. Very recent evidence from cell studies indicates that this could indeed be the case. Romero et al. [30] have shown that the stall force of filopodium retraction strongly depends on the molecular details of filopodium tip adhesion. This result suggests that the proteins located at the filopodium tip, including formins, actively participate in the generation of the pulling forces responsible for retraction. Two other very recent studies in cells [31] , [32] report that cytokinetic ring contraction requires actin depolymerization, and still takes place when myosin motor activity is suppressed. This implies that actomyosin contraction is not the only way to generate mechanical tension in cells. Our findings show that formins anchored to depolymerizing filaments are a molecular alternative to produce the required pulling forces. Proteins and buffers Actin was purified from rabbit muscle. Recombinant Profilin I from mouse was expressed in E. Coli and purified. Spectrin-actin seeds were purified from human erythrocytes. Fluorescent actin was labelled with Alexa488 succinimidyl ester. ADP-actin was made from Ca-ATP-actin, using hexokinase and glucose, converted into Mg-ADP-actin by adding MgCl 2 and EGTA at the beginning of each experiment, and kept on ice for a maximum of 2 h. Formin mDia1(GST-FH1-FH2-DAD-His 6 ), simply referred to as mDia1(FH1FH2), was expressed in E. Coli and purified [9] . Biotinylated mDia1(FH1FH2) was obtained by incubating mDia1(FH1FH2) with either biotinylated anti-His antibody (mouse monoclonal IgG, AnaSpec) or biotinylated anti-GST antibody (mouse monoclonal IgG, Santa Cruz Biotechnology) for at least 1 h on ice. The antibody-to-mDia1FH1FH2 ratio was varied between 0.046 and 2.3 and no differences were observed in the resulting force-velocity curves. Standard elongation and depolymerization of filaments was done in F-buffer (5 mM TRIS pH 7.8, 0.2 mM ATP, 0.1 mM CaCl 2 , 0.01% NaN3, 100 mM KCl, 1 mM MgCl 2 , 0.2 mM EGTA) supplemented with 10 mM DTT and 1 mM DABCO to limit photobleaching. ATP was replaced with ADP+10 μM Ap5A in experiments with ADP-actin. Nucleation of filaments by mDia1(FH1FH2) was carried out at a lower ionic strength, using 50 mM KCl. All measurements were carried out at 25 °C. Sample preparation Glass coverslips were cleaned by sonication in Hellmanex followed by ethanol, rinsed in water and blow dried. Microfluidic chambers were built by assembling clean glass coverslips to PDMS structures composed of three entry channels and one exit channel (more details below). The microchambers were placed on the microscope stage, and connected to the microfluidic system [17] . For control experiments where filament barbed ends grow freely, the microchambers were incubated with spectrin-actin seeds, followed by a solution of BSA. For experiments with anchored mDia1(FH1FH2), the chamber was incubated repeatedly with biotinylated BSA, BSA and Streptavidin, before incubation with biotinylated mDia1(FH1FH2). The specificity of the anchoring of mDia1(FH1FH2) via its biotin tag was tested by flowing mDia1(FH1FH2) pre-incubated with biotinylated antibodies in one half of the microfluidic chamber, and mDia1(FH1FH2) alone in the other half, and verifying that filaments were subsequently nucleated in the region exposed to biotinylated mDia1(FH1FH2) only. The elongation rates of filaments growing from anchored mDia1(FH1FH2) in the absence of mechanical tension were identical to the ones measured on filaments growing from adsorbed spectrin-actin seeds with mDia1(FH1FH2) at their barbed end. Microscopes TIRF and epifluorescence observations were carried out on an Olympus IX71 inverted microscope, with a × 60 TIRF objective, and a 473 nm laser (Cobolt). Images were acquired using a cascade II EMCCD camera (Photometrics). The angles of incidence of the laser beam were determined by mounting a triangular prism on the microscope stage. [33] As the refractive indices of the glass coverslip and buffer solution are known with limited accuracy [33] , we have measured the penetration depth of the TIRF excitation field by monitoring fluorescent microbeads in the flow chamber ( Supplementary Fig. S2 ). The optical trap setup was built on a Nikon eclipse TE2000-U inverted microscope, using an 1064, nm laser, and opto-actoustic deflectors (AA opto-electronics) for attenuation and deflection. Polystyrene microbeads (Polysciences) of 2 μm diameter were used for trapping. The optical trap stiffness was calibrated using the Stokes force on microbeads in a microfluidic flow, and confirmed by the roll-off frequency technique applied in glass microchambers. These measurements were carried out 5 or 10 μm above the coverslip surface, and the same results were obtained at both positions, confirming that the surface was far enough not to perturb these measurements. [34] Images were acquired using an Orca Flash camera (Hamamatsu). Microfluidic system PDMS microchambers were made from photoresist moulds (Stanford Microfluidics Foundry), and mounted on clean glass coverslips. The chambers are composed of three inlets and one outlet. Observations were carried out in the main channel, a few hundred micrometres downstream of the inlets’ junction. The main channel is 1 mm wide and 42 μm high. The flow of solutions in the chamber is controlled and monitored using a MAESFLO system (MFCS and Flowell, from Fluigent). We have verified that the flow rates indicated by the flow metres on the three inlets of our microfluidic apparatus were accurate, within a few per cent. Force calibration and control experiments The friction coefficient of actin filaments was determined using fluorescent filaments growing from spectrin-actin seeds adsorbed on microbeads held in an optical trap, as depicted in Fig. 1a . Force and length were measured within 5 s, for different filament lengths. Force was calibrated for each bead, before growing the filament. The flow velocity at the position of the bead was measured by releasing the bead and monitoring its movement. These measurements allowed us to verify that the force is proportional to filament length times flow velocity, and that the fluctuations of the filament did not bias the measurement. These measurements were repeated at different heights, 5–10 μm above the surface, and in different microchambers, 40–100 μm high, hence with different local flow velocity gradients. This allowed us to verify that the application of a flow velocity gradient had no measurable impact on the force. By monitoring the movement of polystyrene microbeads in the microchamber, we have mapped the velocity profile of the microfluidic flow along the vertical axis. Data were in very good agreement with the theoretical parabolic profile ( Supplementary Fig. S1 ). Thus, the flow profile near the surface is well approximated by a linear function, with a slope that can be computed from the global incoming flow rate and the microchamber dimensions. Using TIRF microscopy, we have taken advantage of the exponential decay of the evanescent excitation field to monitor the vertical position and the fluctuations of the anchored filaments in the fluid flow ( Supplementary Fig. S3 ). These measurements were done on highly labelled filaments (30–70% Alexa488) in order to have a homogeneous fluorescence. We find that fluctuations are larger near the free end of the filament, and larger over the whole filament for lower flow rates. Nevertheless, except for a short region (less than 2 μm long) near the anchoring point, the different portions of the filaments are located 250 nm above the surface on average, and fluctuate within ±30% of this plane. For a given filament profile (that is, a set of z-positions for different portions of the filament), we can compute the force exerted by the flowing fluid on the filament and transmitted to the anchoring point, by integrating the viscous drag exerted on each portion of the filament. We have verified that the result was not affected by the size and number of the filament portions that we considered. By acquiring TIRF images of the fluctuating filament with a high frame rate (down to 17 ms between images) we can monitor the force fluctuations over time. For the present range of flow velocities (up to 200 μm s −1 ) and filament lengths (up to 50 μm), taking the flow velocity 250 nm above the surface and the full-length of the filament reliably gives the average of the force distribution exerted on the anchoring point. Fluctuations are very rapid: the full breadth of the force distribution is explored in less than a second. This ensures that the average force exerted on the anchoring point between two images in our experiments (typically 5 s) is the average force of the distribution. The effect of force fluctuations was estimated by a convolution of the theoretical curves, and found to be negligible. The local flow velocity experienced by surface-anchored filaments was confirmed by exposing highly fluorescent filaments to continuous TIRF illumination in order to fragment them, and monitoring the velocity of detaching fragments with a high camera frame rate. The measured velocities are in good agreement with the height positions estimated by TIRF, with the expected velocity profile near the surface of the flow cell. Control experiments with filaments grown from surface-anchored spectrin-actin seeds were performed in order to measure the elongation and depolymerization rates in the absence of force. These experiments were done with 5–12% Alexa488-labelled G-actin. These experiments also showed that the activity of mDia1(FH1FH2) bound to free barbed ends was not affected by the length of the filament or the microfluidic flow rate. Image analysis Images were analysed using ImageJ. Contrast was enhanced using the KymoToolBox plugin (available from fabrice.cordelieres@curie.upsud.fr). The fluorescent segment of actin filaments was tracked using the ‘snake fit’ programme [35] . Very short fluorescent segments were tracked using the ‘spot tracker 2D′ plugin in Image J (available at http://bigwww.epfl.ch/spottracker/ ). We consider that each actin subunit contributes to 2.7 nm of the filament length. We thus obtained length-versus-time data, which we could fit to extract elongation or depolymerization rates. Knowing the flow rate (measured by the MAESFLO microfluidic apparatus during the experiment) and the length of the filament (full-length, including both the unlabelled and the fluorescently labelled segment), we can compute the force exerted on the surface-anchored mDia1(FH1FH2). How to cite this article: Jégou, A. et al. A Formin mDia1 senses and generates mechanical forces on actin filaments. Nat. Commun. 4:1883 doi: 10.1038/ncomms2888 (2013).